NACA deficiency reveals the crucial role of somite-derived stromal cells in haematopoietic niche formation The ontogeny of haematopoietic niches in vertebrates is essentially unknown. Here we show that the stromal cells of the caudal haematopoietic tissue (CHT), the first niche where definitive haematopoietic stem/progenitor cells (HSPCs) home in zebrafish development, derive from the caudal somites through an epithelial–mesenchymal transition (EMT). The resulting stromal cell progenitors accompany the formation of the caudal vein sinusoids, the other main component of the CHT niche, and mature into reticular cells lining and interconnecting sinusoids. We characterize a zebrafish mutant defective in definitive haematopoiesis due to a deficiency in the nascent polypeptide-associated complex alpha subunit (NACA). We demonstrate that the defect resides not in HSPCs but in the CHT niche. NACA-deficient stromal cell progenitors initially develop normally together with the sinusoids, and HSPCs home to the resulting niche, but stromal cell maturation is compromised, leading to a niche that is unable to support HSPC maintenance, expansion and differentiation. In vertebrate ontogeny, emerging definitive haematopoietic stem/progenitor cells (HSPCs) migrate and colonize successive specialized haematopoietic niches, which in turn regulate proliferation and differentiation of HSPCs, and release of their progeny into the blood. In the most studied haematopoietic niche, the bone marrow of mammals, the cellular constituents so far identified as important for haematopoietic niche function have been endothelial cells of venous sinusoids and arterioles, osteoblasts and associated cells at the endosteal surface, and various stromal cell subsets often closely associated with the blood vessels. Among these are CXCL12-abundant reticular cells [1] , Nestin + perivascular cells [2] , and within the latter subset, Leptin receptor + cells with reticular morphology around venous sinusoids [3] , and NG2 + cells with pericyte morphology around arterioles [4] . The relationship and degree of overlap between these various stromal cell subsets is still to be understood, as well as their relative localization and interaction with HSPCs and with other stromal elements in vivo . In zebrafish development, as in mammals, definitive HSPCs initially emerge by an endothelial-to-haematopoietic transition from the ventral wall (‘floor’) of the dorsal aorta (VDA) [5] , and then migrate through the blood to colonize the first niche where they will expand and differentiate into multiple blood lineages. In fish, this initial niche is the caudal haematopoietic tissue (CHT [6] , [7] ), while in mammals it is the fetal liver. The fetal liver haematopoietic niche is still poorly characterized [8] . We previously reported that the CHT of zebrafish is organized around a transient network of venous sinusoids, the caudal vein (CV) plexus, and that its ultrastructural organization is quite similar to the peri-sinusoidal haematopoietic microenvironment in the haematopoietic niche of adults—the bone marrow in mammals, or the kidney marrow in fish—with typical fibroblastic reticular cells (FRCs) in close contact with the abluminal side of venous sinusoids and extending a network between the latter, within which haematopoietic cells expand and differentiate [6] . In the CHT, these FRCs appear to be the main stromal cell type making up the niche together with the endothelium of the CV plexus/sinusoids. Thanks to the transparency of the zebrafish larva, the CHT is uniquely accessible to non invasive in vivo observation, offering a unique opportunity to explore in situ the development of this haematopoietic niche at a cellular level. In the present study, we show that the stromal FRCs of the CHT niche derive from the ventral border of the caudal somites, through an epithelial–mesenchymal transition (EMT). We find that a deficiency in the α-subunit of the nascent polypeptide-associated complex (NACA, αNAC) prevents the maturation of the EMT-derived mesenchymal progenitors of the FRCs, and that this results in a CHT niche that can still trap circulating HSPCs, but is no longer able to retain them and support their expansion and differentiation. The NACA-deficient mutant thus highlights the essential role of these stromal FRCs in the making of a functional haematopoietic niche. The oloca mutant is defective in definitive haematopoiesis We identified the zebrafish mutant oloca as a recessive mutant with fewer neutrophils by 3.5–4 days post fertilization (d.p.f. ), using Sudan Black (SB) staining in a F3 mutant screen following ENU mutagenesis. SB staining of the oloca mutant showed fewer neutrophils in the head ( Fig. 1b ), and no neutrophils in the CHT ( Fig. 1d ), which normally produces numerous neutrophils by this stage [9] ( Fig. 1a,c ). The few SB + cells found in the oloca tail were not localized within the CHT but at the body surface ( Fig. 1d , arrows). Oloca mutants develop apparently normally up to 2.5–3 d.p.f. Morphological defects become obvious after 3.5 d.p.f. : a small head with immature lower jaw, cardiac oedema, disorganized iridophores in eyes, reduced circulation from 90 h post fertilization (h.p.f.) onward, and finally the larvae die by ∼ 4.5 d.p.f. 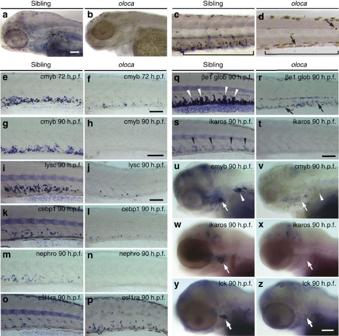Figure 1: Definitive haematopoiesis is defective in theolocamutant. (a–d) Sudan black (SB) staining of sibling andolocamutant at 3.5 d.p.f. in the rostral (a,b) and caudal (CHT;c,d) area. Arrows in (d) indicate SB+cells located outside of the CHT. Brown spots are pigment cells. (e–z) Whole-mountin situhybridization using indicated probes inolocaand sibling larvae. (e–h)cmybat 72 and 90 h.p.f. (i–p)lysozyme c,c/ebp 1,nephrosinandcsf1raat 90 h.p.f. (q,r)βE1-globinat 90 h.p.f.. White arrowheads and black arrows indicate definitive haematopoietic clusters and circulating primitive erythrocytes, respectively. (s,t)ikarosat 90 h.p.f.; arrowheads indicate definitive haematopoietic clusters. (u–z)cmyb,ikarosandlckat 90 h.p.f.; arrows and arrowheads indicate thymus and kidney, respectively. Non-specific signal is seen in the notochord in panels (i,k,o,q,s). Scale bars, 100 μm. Figure 1: Definitive haematopoiesis is defective in the oloca mutant. ( a – d ) Sudan black (SB) staining of sibling and oloca mutant at 3.5 d.p.f. in the rostral ( a , b ) and caudal (CHT; c , d ) area. Arrows in ( d ) indicate SB + cells located outside of the CHT. Brown spots are pigment cells. ( e – z ) Whole-mount in situ hybridization using indicated probes in oloca and sibling larvae. ( e – h ) cmyb at 72 and 90 h.p.f. ( i – p ) lysozyme c , c/ebp 1 , nephrosin and csf1ra at 90 h.p.f. ( q , r ) βE1-globin at 90 h.p.f.. White arrowheads and black arrows indicate definitive haematopoietic clusters and circulating primitive erythrocytes, respectively. ( s , t ) ikaros at 90 h.p.f. ; arrowheads indicate definitive haematopoietic clusters. ( u – z ) cmyb , ikaros and lck at 90 h.p.f. ; arrows and arrowheads indicate thymus and kidney, respectively. Non-specific signal is seen in the notochord in panels ( i , k , o , q , s ). Scale bars, 100 μm. Full size image As the SB phenotype suggested a lack of definitive granulopoiesis in the CHT of oloca larvae, we analysed the status of definitive haematopoiesis in the CHT by whole mount in situ hybridization (WISH). At 72 h.p.f., much fewer cmyb + HSPCs were found in the oloca CHT compared with siblings ( Fig. 1e,f ), and none at all from 90 h.p.f. onwards ( Fig. 1g,h ). Accordingly, by 90 h.p.f., granulopoiesis, probed by lysC , cebp1 and nephrosin expression ( Fig. 1i–n ), erythropoiesis, probed by ße1-globin expression ( Fig. 1q,r ), and lymphopoiesis probed by ikaros expression ( Fig. 1s,t ) were all strongly reduced. The final definitive haematopoietic tissues, the thymus and kidney, which normally become seeded by HSPCs from the CHT by 3 and 5 d.p.f. respectively [6] , similarly lacked cmyb expression in oloca embryos ( Fig. 1u,v ), and the lymphoid markers ikaros and lck were missing in the mutant thymus ( Fig. 1w–z ). In contrast with the other haematopoietic lineages, csf1ra expression, which marks the macrophage lineage, was similar to siblings or even slightly increased in the CHT of oloca mutants ( Fig. 1o,p ). This is consistent with our observations that primitive macrophages, born in the yolk sac, colonize the nascent CHT through blood circulation before definitive haematopoiesis takes place there [6] . Oloca is a mutant in the naca gene To identify the mutation responsible for the oloca phenotype, we used simple sequence length polymorphism mapping. The mutation was mapped between flanking markers z7590 and w27205 ( Fig. 2a ) on chromosome 23. This interval is ∼ 450 kb and contains around 20 genes. One of them, naca , had been previously identified in an insertional mutagenesis screen as no knack [10] . no knack is an essential gene and the terminal phenotype was similar to oloca . In a cross with oloca , no knack failed to complement, strongly suggesting that oloca was a naca mutant. Sequencing of the zebrafish naca gene, in mutant and sibling embryos, revealed a premature stop codon in the mutant allele due to a C→T transition, resulting in a Q>stop alteration at codon 69 ( Fig. 2b,c ). The naca gene encodes the α subunit of the heterodimeric nascent polypeptide-associated complex (αNAC/NACA), which binds to nascent polypeptides on the ribosome [11] . NACA appears to be part of the chaperon system that ensures the proper folding of nascent proteins, notably those to be translocated in the endoplasmic reticulum, ER [12] , [13] . The naca gene also encodes a muscle-specific, much larger isoform, skNAC, through differential RNA splicing [14] , [15] . NACA and skNAC have also been described as transcriptional co-activators in osteoblasts and myotubes, respectively [14] , [16] , [17] . 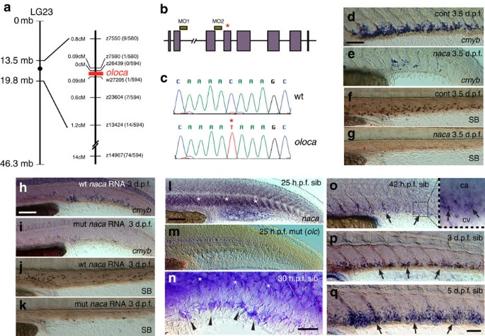Figure 2: Genetic characterization of theolocamutant. (a) Mapping of theolocamutation using co-segregation of known simple sequence length polymorphism markers;olocawas located between w27205 and z7590 on linkage group (LG) 23. (b,c) Thenacagene contains 8 exons and a C-to-T substitution was found in exon 4 in the mutant (asterisk). Splice-blocking MOs MO1 and MO2 were designed at the positions indicated. (d–g) wild-type embryos were injected with 4 ng of control ornacaMO1 and analysed by WISH using acmybprobe and by SB staining at 3.5 d.p.f. (h–k) Co-injection ofnacaMO1 with 125 pg of wild-type or mutantnacaRNA and subsequent analysis of the caudal area at 3 d.p.f. as in (d–g). (l–q) WISH fornacaexpression in the caudal area from 1 to 5 d.p.f. White asterisks show the stronger expression ofnacain the ventral half of somites at 25 and 30 h.p.f. in the siblings (l,n), while no signal is detected in the mutant embryos (m). Arrowheads in (n) indicate the first, mesenchymal-shaped cells expressingnacain the nascent CHT at 30 h.p.f. At 42 h.p.f.,nacaexpression has greatly diminished in the somites and is mostly observed in the CHT in a small cell population (arrows and inset), that becomes much larger by 3 and 5 d.p.f. (p,q). ca, caudal artery; cv, definitive caudal vein (ventral-most branch of the CV plexus). Scale bars, 100 μm (d,h,l) and 50 μm (n,q). Figure 2: Genetic characterization of the oloca mutant. ( a ) Mapping of the oloca mutation using co-segregation of known simple sequence length polymorphism markers; oloca was located between w27205 and z7590 on linkage group (LG) 23. ( b , c ) The naca gene contains 8 exons and a C-to-T substitution was found in exon 4 in the mutant (asterisk). Splice-blocking MOs MO1 and MO2 were designed at the positions indicated. ( d – g ) wild-type embryos were injected with 4 ng of control or naca MO1 and analysed by WISH using a cmyb probe and by SB staining at 3.5 d.p.f. ( h – k ) Co-injection of naca MO1 with 125 pg of wild-type or mutant naca RNA and subsequent analysis of the caudal area at 3 d.p.f. as in ( d – g ). ( l – q ) WISH for naca expression in the caudal area from 1 to 5 d.p.f. White asterisks show the stronger expression of naca in the ventral half of somites at 25 and 30 h.p.f. in the siblings ( l , n ), while no signal is detected in the mutant embryos ( m ). Arrowheads in ( n ) indicate the first, mesenchymal-shaped cells expressing naca in the nascent CHT at 30 h.p.f. At 42 h.p.f., naca expression has greatly diminished in the somites and is mostly observed in the CHT in a small cell population (arrows and inset), that becomes much larger by 3 and 5 d.p.f. ( p , q ). ca, caudal artery; cv, definitive caudal vein (ventral-most branch of the CV plexus). Scale bars, 100 μm ( d , h , l ) and 50 μm ( n , q ). Full size image To provide independent evidence that the naca mutation causes the oloca phenotype, we tested whether morpholinos (MOs) targeted against naca RNA would phenocopy the oloca mutant, and whether wild-type naca RNA injection would rescue the oloca phenotype. Two naca splice-blocking MOs, MO1 and MO2, phenocopied the oloca mutant. In the CHT of naca MO1-injected embryos, very few cmyb -positive HSPCs and almost no SB stained neutrophil were observed at 3.5 d.p.f. ( Fig. 2d–g ). Co-injection of 125 or 250 pg of naca wild-type RNA with 4 ng of naca MO1 resulted in rescue of cmyb + HSPCs and neutrophil differentiation (SB staining) in the naca morphants ( Fig. 2h,j ). In contrast, co-injection of the same amounts of naca mutant RNA with naca MO1 did not rescue the morphant phenotype to any extent ( Fig. 2i,k ). WISH analysis through development revealed ubiquitous expression of naca mRNA at 25–30 h.p.f., with a stronger signal in the ventral half of somites ( Fig. 2l , asterisks) and in mesenchymal cells ventral to the somites in the caudal area ( Fig. 2n , arrowheads). By 3 and 5 d.p.f. (by which stage haematopoiesis peaks in the CHT), naca has become specifically expressed in the CHT ( Fig. 2p,q , arrows), a trend that appears to initiate by 42 h.p.f. ( Fig. 2o , arrows). In oloca mutant embryos, WISH detected no naca transcripts, suggesting nonsense mediated mRNA decay ( Fig. 2m ). HSPCs initially home to the mutant CHT We used naca MO1 to assess the early effects of NACA deficiency on haematopoiesis, at stages at which mutant embryos cannot yet be distinguished morphologically. naca MO1-injected embryos showed normal primitive haematopoiesis, including granulopoiesis of yolk sac origin ( Supplementary Fig. 1 , arrows), and erythrocyte circulation. By 36 h.p.f., cmyb -positive definitive HSPCs were found along the aorta ventral wall (VDA) and nascent CHT of naca morphant embryos as in wild type ( Fig. 3a,b ). To follow their fate in live embryos, we turned to transgenic Tg[CD41:gfp] embryos, as definitive HSPCs are CD41:GFP low from as soon as they emerge from the VDA [18] (from here onwards, gfp will refer to the transgene, and, for example, CD41:GFP to the fluorescence of the GFP protein expressed from the CD41:gfp transgene). Consistently, naca MO1-injected Tg[CD41:gfp] embryos showed normal emergence of CD41:GFP low HSPCs from the VDA at 54 h.p.f. ( Fig. 3c,d,k ) and their settling in the CHT ( Fig. 3e,f,k ). Thus, definitive HSPCs were normally specified and produced from the morphant DA floor (VDA), and initially colonized the CHT as in wild type. 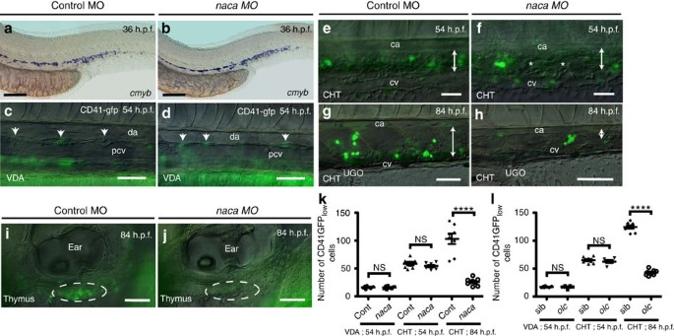Figure 3: Definitive, aorta-derived HSPCs home to the CHT niche but fail to proliferate and differentiate there innacamorphants and mutants. (a–k) Tg[CD41:gfp] embryos were injected with control ornacaMOs. (a,b) Expression ofcmybat 36 h.p.f. marking HSPC emergence in control (a) andnacamorphant (b) embryos. (c–j)in vivocombined VE-DIC/fluorescence microscopy of control (c,e,g,i) andnacaMO-injected embryos (d,f,h,j). (c,d) Arrows indicate emergence of CD41:GFPlowHSPCs along the VDA at 54 h.p.f. (e,f) Colonization of the CHT by CD41:GFPlowHSPCs is seen in both control and morphant embryos at 54 h.p.f. The thickness of CV plexus is almost the same between control and morphant embryos (double arrows). CV plexus segments devoid of any haematopoietic cells were observed in the morphant CHT only (f, asterisks). (g,h) At 84 h.p.f., the CHT has become much thinner in the morphant (h, double arrow) and the number of CD41-GFPlowHSPCs and CD41-GFPhighprothrombocytes is much lower. (i,j) At 84 h.p.f., no CD41-GFPlowlymphoid progenitors were detected in the morphant thymus (j, dotted circle), unlike in control larvae (i). Number of CD41:GFPlowcells in the VDA (at 54 h.p.f.) and CHT (54 and 84 h.p.f.) of control ornacaMO-injected (k), andoloca[CD41:gfp] sibling and mutant (l) embryos (mean±s.d.,n=2 separate experiments). Statistical significance determined using a Student’st-test. ****P<0.0001. n.s., not significant. cv, caudal vein; ca, caudal artery; pcv, posterior cardinal vein; da, dorsal aorta; UGO, uro-genital opening. Scale bars, 100 μm (a,b) and 50 μm (c–j). Figure 3: Definitive, aorta-derived HSPCs home to the CHT niche but fail to proliferate and differentiate there in naca morphants and mutants. ( a – k ) Tg[CD41:gfp] embryos were injected with control or naca MOs. ( a , b ) Expression of cmyb at 36 h.p.f. marking HSPC emergence in control ( a ) and naca morphant ( b ) embryos. ( c – j ) in vivo combined VE-DIC/fluorescence microscopy of control ( c , e , g , i ) and naca MO-injected embryos ( d , f , h , j ). ( c , d ) Arrows indicate emergence of CD41:GFP low HSPCs along the VDA at 54 h.p.f. ( e , f ) Colonization of the CHT by CD41:GFP low HSPCs is seen in both control and morphant embryos at 54 h.p.f. The thickness of CV plexus is almost the same between control and morphant embryos (double arrows). CV plexus segments devoid of any haematopoietic cells were observed in the morphant CHT only ( f , asterisks). ( g , h ) At 84 h.p.f., the CHT has become much thinner in the morphant ( h , double arrow) and the number of CD41-GFP low HSPCs and CD41-GFP high prothrombocytes is much lower. ( i , j ) At 84 h.p.f., no CD41-GFP low lymphoid progenitors were detected in the morphant thymus ( j , dotted circle), unlike in control larvae ( i ). Number of CD41:GFP low cells in the VDA (at 54 h.p.f.) and CHT (54 and 84 h.p.f.) of control or naca MO-injected ( k ), and oloca [CD41:gfp] sibling and mutant ( l ) embryos (mean±s.d., n =2 separate experiments). Statistical significance determined using a Student’s t -test. **** P <0.0001. n.s., not significant. cv, caudal vein; ca, caudal artery; pcv, posterior cardinal vein; da, dorsal aorta; UGO, uro-genital opening. Scale bars, 100 μm ( a , b ) and 50 μm ( c – j ). Full size image In contrast, 30 h later, by 84 h.p.f., the morphant CHT contained much less CD41:GFP low HSPCs than control embryos ( Fig. 3g,h,k ). This decline in HSPC number in the morphant CHT was accompanied by a strong reduction in the dorso-ventral width of the CHT. In addition, whereas CD41:GFP low lymphoid progenitors normally start colonizing the thymus rudiment from 54 h.p.f. onwards [18] , the naca morphant thymus rudiment showed no such colonization even at 84 h.p.f. ( Fig. 3i,j ), consistent with our previous WISH data with the oloca mutant ( Fig. 1u–z ). Thus NACA deficiency did not affect HSPC emergence from the aorta, nor their initial homing in the CHT, but their subsequent maintenance, expansion and differentiation in the CHT. The same outcomes were observed with oloca :CD41gfp mutant embryos ( Fig. 3l ). The mutant CHT niche is unable to support HSPC development To analyse whether the defect of definitive haematopoiesis in the mutant CHT is cell-autonomous or non-cell-autonomous, we transplanted wild-type CMTPX-labelled whole kidney marrow (WKM) cells from adult Tg[mpx:gfp] fish, or GFP + neutrophils sorted from the WKM preparation, into the sinus venosus of non-transgenic oloca mutant and sibling embryos at 48 h.p.f., and we followed up their fate in the live larvae. 1.5–2.5 h post transplantation (h.p.t. ), many CMTPX-stained WKM or mpx:GFP + transplanted cells had already homed to the CHT plexus and to the pronephric kidney area in both sibling and mutant embryos ( Fig. 4a and Supplementary Fig. 2a–d ). By 7 h.p.t., virtually all transplanted cells had settled in the haematopoietic tissues, in similar amounts in mutant and sibling embryos. Then in the resulting sibling larvae, the adult CMPTX + WKM cells remained in the CHT and kidney area, and by 30 h.p.t. (78 h.p.f. ), they had already strongly expanded there ( Fig. 4b,c ). In sharp contrast, in the mutant recipient larvae, CMTPX + cells were no longer observed in the CHT and very few transplanted cells were detected in the kidney area by this stage ( Fig. 4b,d ). The same outcome occurred with the transplanted mpx:GFP + adult WKM-derived neutrophils that homed to the CHT. In the sibling larvae, by 36 h.p.t. they were still in the CHT and kidney area ( Supplementary Fig. 2e,g , Supplementary Movie 1 ) where they had expanded, and some were seen undergoing mitosis (as commonly observed also with endogenous larval mpx:GFP + neutrophils). In contrast, in the mutant larvae, the transplanted mpx:GFP + cells, which had similarly homed to the CHT up to 7 h.p.t., started leaving it from 12 h.p.t. onwards, entering circulation as well as migrating into surrounding superficial tissues, such that by 36 h.p.t., very few mpx:GFP + cells were remaining in the CHT and kidney area ( Supplementary Fig. 2f,h , Supplementary Movie 1 ). TUNEL staining on the recipient mutant larvae confirmed that the transplanted mpx:GFP + cells that initially homed to the CHT did not disappear by apoptosis. 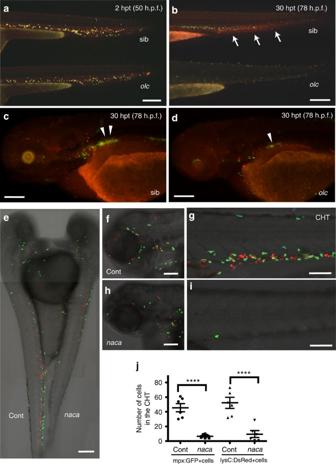Figure 4:nacais non-cell autonomously required for HSPC settlement and proliferation/differentiation in the CHT. (a) Fluorescence microscopy of sibling andolocamutant transplanted at 48 h.p.f. with CMTPX-stained WKM cells obtained from adult Tg[mpx:gfp] fish. Numerous mpx:GFP+(green) and/or CMTPX+(red) WKM cells were observed in the CHT niche of botholocamutant (olc) and sibling embryos at 2 h post transplantation (h.p.t.=50 h.p.f.). (b) Almost no remaining transplanted cells were detected in the CHT ofolcembryo at 30 h.p.t. whereas CMTPX+WKM cells had expanded in the sibling CHT (arrows). (c,d) In the kidney area, stable colonization of transplanted WKM cells was detected in the sibling larva whereas very few transplanted cells were observed in theolcembryo at 30 h.p.t. (arrowheads). (e–i) Confocal microscopy analysis at 60 h.p.f. of parabiotic embryo pairs composed of a control MO-injected Tg[lysC:DsRed] embryo and anacaMO-injected Tg[mpx:gfp] embryo. A parabiotic pair is shown in (e), and magnified images of the head (f,h) and CHT (g,i) of both parabiotic partners are shown. (j) For six such parabiotic pairs, the number of GFP+and DsRed+cells was counted in the CHT of both partners (‘cont’ and ‘naca’, mean±s.d.;n=3 separate experiments). Scale bars, 200 μm (a,b,e), 150 μm (c,d) and 100 μm (f–i). Statistical significance determined using a Student’st-test. ****P<0.0001. Figure 4: naca is non-cell autonomously required for HSPC settlement and proliferation/differentiation in the CHT. ( a ) Fluorescence microscopy of sibling and oloca mutant transplanted at 48 h.p.f. with CMTPX-stained WKM cells obtained from adult Tg[mpx:gfp] fish. Numerous mpx:GFP + (green) and/or CMTPX + (red) WKM cells were observed in the CHT niche of both oloca mutant ( olc ) and sibling embryos at 2 h post transplantation (h.p.t.=50 h.p.f.). ( b ) Almost no remaining transplanted cells were detected in the CHT of olc embryo at 30 h.p.t. whereas CMTPX + WKM cells had expanded in the sibling CHT (arrows). ( c , d ) In the kidney area, stable colonization of transplanted WKM cells was detected in the sibling larva whereas very few transplanted cells were observed in the olc embryo at 30 h.p.t. (arrowheads). ( e – i ) Confocal microscopy analysis at 60 h.p.f. of parabiotic embryo pairs composed of a control MO-injected Tg[lysC:DsRed] embryo and a naca MO-injected Tg[mpx:gfp] embryo. A parabiotic pair is shown in ( e ), and magnified images of the head ( f , h ) and CHT ( g , i ) of both parabiotic partners are shown. ( j ) For six such parabiotic pairs, the number of GFP + and DsRed + cells was counted in the CHT of both partners (‘cont’ and ‘ naca ’, mean±s.d. ; n =3 separate experiments). Scale bars, 200 μm ( a , b , e ), 150 μm ( c , d ) and 100 μm ( f – i ). Statistical significance determined using a Student’s t -test. **** P <0.0001. Full size image HSPCs are not intrinsically compromised in the oloca mutant We next addressed whether the haematopoietic defect in the oloca mutant was solely due to its deficient CHT niche, or whether it also involved a cell-autonomous defect of mutant HSPCs. To address this point, we took advantage of a recent method for generating parabiotic embryo pairs [19] , applying it to Tg[mpx:gfp] and Tg[lysC:DsRed] embryos, that give rise to green and red fluorescent neutrophils, respectively. When we generated parabiotic wild-type Tg[mpx:gfp]/Tg[lysC:DsRed] embryo pairs, by 60 h.p.f., the CHTs of both embryos displayed both GFP + and DsRed + neutrophils, indicating that the definitive HSPCs born from the aortas of both embryos had similarly homed to both CHTs and given rise to (resp. GFP + and DsRed + ) neutrophils ( Supplementary Fig. 2i–m ). We then performed the same parabiosis experiment but using naca MO-injected Tg[mpx:gfp] and control MO-injected Tg[lysC:DsRed] partner embryos ( Fig. 4e ). By 60 h.p.f., mpx:GFP + and lysC:DsRed + cells were similarly observed in the rostral region of both control and naca MO-injected embryos ( Fig. 4f,h ), consistent with the unimpaired primitive granulopoiesis in naca mutants. In contrast, numerous mpx:GFP + and lysC:DsRed + cells were observed in the CHT of control MO-injected lysC:DsRed embryos whereas only few cells of either origin were found in the naca morphant CHT ( Fig. 4g,i,j ). These results confirm that naca deficiency leads to a deficient CHT niche and show that, in contrast, the homing capacity and granulocytic differentiation ability of NACA-deficient definitive HSPCs is intact. CHT stromal cells originate from the caudal somites In our initial description of the CHT niche [6] , our electron microscopy data suggested it to consist in two main cell types, the endothelial cells of the CV plexus sinusoids, and mesenchymal cells in between the sinusoids that appeared to evolve into what we called FRCs, owing to their ultrastructural resemblance to FRCs in mammalian bone marrow and adult fish kidney marrow. Therefore we screened various existing transgenic reporters in search of one that would highlight the FRCs and their progenitors. We found that a pair of Wnt signalling reporter lines, Tg[TCF:nls-mCherry] and Tg[TCF:gfp] [20] , respectively expressing nuclear mCherry and whole-cell GFP, appeared to do so. As previously described [20] , by 20 h.p.f. (24-somites), these two reporters are highly expressed in the caudal somites. Time-lapse confocal imaging of Tg[TCF:gfp] embryos from 21 h.p.f. revealed that TCF:GFP + cells belonging to the ventral side of the caudal somites started to migrate ventrally, and settled in the future CHT by 25–28 h.p.f. ( Supplementary Fig. 3a and Supplementary Movie 2 ). The same cells and migration pattern were revealed using Tg[TCF:nls-mCherry] embryos ( Supplementary Movie 3a ). We thus combined the time-lapse confocal imaging of the TCF:nls-mCherry + nuclei of these emigrating cells with vital staining with the interstitial fluorescent marker Bodipy ceramide, which has been used to delineate somite and cell contours within the somitic epithelium [21] , [22] ( Supplementary Fig. 3b ). The four-dimensional tracking of individual nuclei of the emigrating cells confirmed that they were initially all intra-somitic, and located within the entire medio-lateral extent of the ventral border of the somites ( Supplementary Fig. 3c–e and Supplementary Movie 4 ). We studied this emigration process in more detail by combining fluorescence with video-enhanced Differential Interference Contrast (VE-DIC) microscopy [6] . From 19 h.p.f., epithelial cells from the ventral part of the caudal somites underwent an EMT. They started to show active blebbing through the somite basal lamina ( Fig. 5a and Supplementary Movie 5 ), then more extended protrusions in ventral direction ( Fig. 5b ), and emigrated as strings of mesenchymal cells into the more ventral caudal space, with frequent mitoses before and during their migration ( Fig. 5c–e , Supplementary Movie 6 ). In that space, at the same time, the primordial CV started sprouting in ventral direction to give rise to the CV plexus by 30 h.p.f. To observe the interaction between the two processes, we crossed Tg[TCF:nls-mCherry] with Tg[fli1:gfp] fish. At 25 h.p.f., the angiogenic sprouting of endothelial cells from the primordial CV was very dynamic, and TCF:nls-mcherry + cells were found interspersed with the endothelial sprouts ( Supplementary Movie 3b ), interacting with them and with each other through filopodial extensions ( Fig. 5f,g ). By 35 h.p.f., the CV plexus was complete and functional [6] . Between 35 and 48 h.p.f., the cytomorphology and distribution of nls-mCherry + mesenchymal cells in the CHT evolved. By 35 h.p.f. they displayed a large nucleus, scant cytoplasm and long filopodia by which they connected to each other and to endothelial cells ( Fig. 5i,j ). By 48 h.p.f., their nuclei had become smaller, with a central, well-defined nucleolus, and while they were still making a dynamic network of interconnecting filopodial extensions connecting them to each other and other cells ( Fig. 5k and Supplementary Movie 7 ), many of them now had their cell body in close apposition to the abluminal side of endothelial cells of the CV plexus ( Fig. 5h,l ). This configuration is identical to that of the FRCs that we previously described by electron microscopy as the main stromal cell type making up the CHT niche together with the endothelial cells of the CV plexus [6] . We further evidenced the somitic origin of these cells by transiently expressing GFP from a skeletal muscle α-actin promoter in Tg[TCF:nls-mCherry] embryos. By 22 h.p.f., [GFP + ; nls-mCherry + ] double positive cells were observed throughout the somites ( Supplementary Fig. 4a–c ). Then double-positive cells were observed by 24 h.p.f. emigrating from the somites ( Supplementary Fig. 4d–f ), and by 36 h.p.f. among the developing stromal cells both between and in close apposition to the CV plexus endothelia ( Supplementary Fig. 4g–m ) as previously observed ( Fig. 5h,l ). 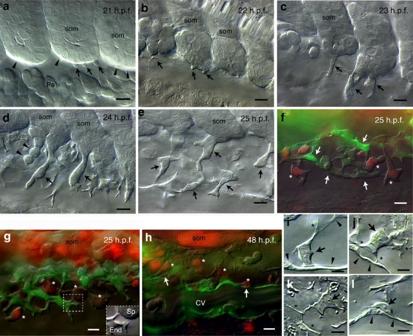Figure 5: Ontogeny of stromal progenitors and interaction with endothelial cells of the developing CV plexus. in vivoobservation of [TCF:nls-mCherry; Fli1:gfp] double transgenic embryos. (a–e) VE-DIC microscopy reveals the epithelial–mesenchymal transition giving rise to stromal progenitors. (a) Active cell blebbing (arrows andSupplementary Movie 5) through the somite basal lamina (arrowheads) was often observed at the ventral side of caudal somite epithelial cells by 21 h.p.f. (b) An hour later (22 h.p.f.), the transient blebs were replaced by more stable protrusions (arrows), then the cells started to emigrate from the somite as mesenchymal cells (c,d); mitosis was often observed around the onset of this emigration (d, arrowheads), and the emigrating cells tended to form strings (e, arrows) and interact through filopodia. (f,g) By the same stage (25 h.p.f.), VE-DIC and fluorescence overlay shows physical interactions between these nls-mCherry+stromal cell progenitors (asterisks) and the Fli1:GFP+endothelial cells of the developing CV plexus (f, arrows); the inset in (g) shows such an interaction at higher magnification. (h) One day later, among the nls-mCherry+stromal cells (asterisks), some have now settled in adventitial position (arrows) along the endothelial cells forming the main caudal vein. (i–l) VE-DIC imaging of the cytomorphological maturation of stromal progenitors in relation to the CV plexus. (i,j) At 36 h.p.f., young stromal progenitors display a large nucleus (arrows) and interact with endothelial cells (arrowheads) through their filopods (asterisks). (k,l) At 48 h.p.f., two types of TCF:nls-mCherry+stromal cells are observed; interconnecting (k) and adventitial (l) stromal cells. Nucleoli were often clearly visible in those stromal cells at this stage (arrows). Arrowheads and asterisks indicate endothelial cells and filopods of stromal cells, respectively. som, somite; sp, stromal progenitor; end, endothelial cell; cv, caudal vein. Scale bars, 10 μm (a–h) and 5 μm (i–l). Figure 5: Ontogeny of stromal progenitors and interaction with endothelial cells of the developing CV plexus. in vivo observation of [TCF:nls-mCherry; Fli1:gfp] double transgenic embryos. ( a – e ) VE-DIC microscopy reveals the epithelial–mesenchymal transition giving rise to stromal progenitors. ( a ) Active cell blebbing (arrows and Supplementary Movie 5 ) through the somite basal lamina (arrowheads) was often observed at the ventral side of caudal somite epithelial cells by 21 h.p.f. ( b ) An hour later (22 h.p.f. ), the transient blebs were replaced by more stable protrusions (arrows), then the cells started to emigrate from the somite as mesenchymal cells ( c , d ); mitosis was often observed around the onset of this emigration ( d , arrowheads), and the emigrating cells tended to form strings ( e , arrows) and interact through filopodia. ( f , g ) By the same stage (25 h.p.f. ), VE-DIC and fluorescence overlay shows physical interactions between these nls-mCherry + stromal cell progenitors (asterisks) and the Fli1:GFP + endothelial cells of the developing CV plexus ( f , arrows); the inset in ( g ) shows such an interaction at higher magnification. ( h ) One day later, among the nls-mCherry + stromal cells (asterisks), some have now settled in adventitial position (arrows) along the endothelial cells forming the main caudal vein. ( i – l ) VE-DIC imaging of the cytomorphological maturation of stromal progenitors in relation to the CV plexus. ( i , j ) At 36 h.p.f., young stromal progenitors display a large nucleus (arrows) and interact with endothelial cells (arrowheads) through their filopods (asterisks). ( k , l ) At 48 h.p.f., two types of TCF:nls-mCherry + stromal cells are observed; interconnecting ( k ) and adventitial ( l ) stromal cells. Nucleoli were often clearly visible in those stromal cells at this stage (arrows). Arrowheads and asterisks indicate endothelial cells and filopods of stromal cells, respectively. som, somite; sp, stromal progenitor; end, endothelial cell; cv, caudal vein. Scale bars, 10 μm ( a – h ) and 5 μm ( i – l ). Full size image Finally, in vivo observation of Tg[sox10:gfp] which highlights neural crest cells (NCCs) [23] , revealed no NCC contribution to the CHT other than pigment cells ( Supplementary Fig. 5a,c ). Moreover, sox10 mutants lacking most NCC derivatives revealed no sox10:GFP + cells in the CHT, yet no morphological abnormality of the CHT, and the presence of typical stromal cells as in the wild type ( Supplementary Fig. 5a–h ), indicating that NCCs do not contribute to stromal cell development during CHT niche formation. We therefore conclude that the FRCs/stromal cells initially arise from the caudal somites through a typical EMT, and that their progenitors accompany the formation of the CV plexus, leading altogether to the final haematopoietic niche. From now on, we will designate these cells as stromal cells or stromal reticular cells (SRCs). Naca is required for stromal cell maturation We next compared the development of caudal endothelial (Fli1:GFP + ) and stromal (TCF:nls-mCherry + ) cells between control and naca morphant embryos. Time-lapse confocal analysis on [Fli1:gfp; TCF:nls-mCherry] double transgenic embryos indicated that the initial sprouting of Fli1:GFP + CV endothelial cells and parallel emigration of TCF:nls-mCherry + stromal cell progenitors from the somites occurred normally in morphant embryos compared with controls ( Fig. 6a,b ). 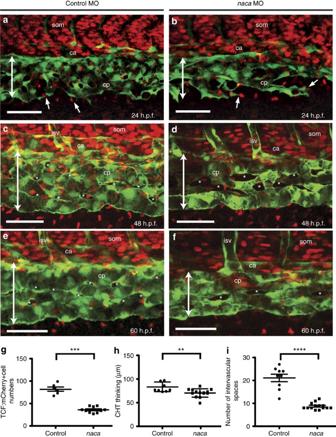Figure 6: Stromal cells gradually disappear in the CHT of NACA-depleted embryos. (a–f) Live confocal fluorescence imaging of the CHT area in control andnacaMO-injected [TCF:nls-mCherry; Fli1:gfp] double transgenic embryos at 24, 48 and 60 h.p.f. Double arrows indicate the thickness of the developing CV plexus. (a,b) Arrows indicate some of the stromal cell progenitors accompanying the protrusion of Fli1:GFP+endothelial cells sprouted from the primordial CV. (c–f) Asterisks indicate intervascular spaces within the CV plexus; note that these spaces in the morphant (d) are larger and flatter at 48 h.p.f. than in control embryo (c), and that they contain fewer nls-mCherry+stromal cells at 48 h.p.f., and virtually none at 60 h.p.f. (f). (g) Number of TCF:nls-mCherry+cells in the CHT of control andnacaMO-injected embryos at 48 h.p.f. Six control and 10nacaMO-injected embryos were analysed. (h,i) Comparison of the thickness (h) and number of intervascular spaces (i) of the CV plexus between control andnacamorphant embryos at 48 h.p.f. Nine control and 14nacaMO-injected embryos were analysed. Error bars represent the s.d. Statistical significance determined using a Student’st-test. **P<0.01; ***P<0.001; ****P<0.0001. som, somite; ca, caudal artery; cp, caudal vein plexus; isv, inter-somitic vessel. Scale bars, 50 μm. Figure 6: Stromal cells gradually disappear in the CHT of NACA-depleted embryos. ( a – f ) Live confocal fluorescence imaging of the CHT area in control and naca MO-injected [TCF:nls-mCherry; Fli1:gfp] double transgenic embryos at 24, 48 and 60 h.p.f. Double arrows indicate the thickness of the developing CV plexus. ( a , b ) Arrows indicate some of the stromal cell progenitors accompanying the protrusion of Fli1:GFP + endothelial cells sprouted from the primordial CV. ( c – f ) Asterisks indicate intervascular spaces within the CV plexus; note that these spaces in the morphant ( d ) are larger and flatter at 48 h.p.f. than in control embryo ( c ), and that they contain fewer nls-mCherry + stromal cells at 48 h.p.f., and virtually none at 60 h.p.f. ( f ). ( g ) Number of TCF:nls-mCherry + cells in the CHT of control and naca MO-injected embryos at 48 h.p.f. Six control and 10 naca MO-injected embryos were analysed. ( h , i ) Comparison of the thickness ( h ) and number of intervascular spaces ( i ) of the CV plexus between control and naca morphant embryos at 48 h.p.f. Nine control and 14 naca MO-injected embryos were analysed. Error bars represent the s.d. Statistical significance determined using a Student’s t -test. ** P <0.01; *** P <0.001; **** P <0.0001. som, somite; ca, caudal artery; cp, caudal vein plexus; isv, inter-somitic vessel. Scale bars, 50 μm. Full size image By 48 h.p.f., about two times less TCF:nls-mCherry + stromal cells were detected in the naca morphant CHT relative to controls ( Fig. 6c,d,g ). However this did not necessarily reflect a true decrease in stromal cell number at this stage, because the mean mCherry fluorescence per detected cell was also diminished over 2-fold in both the somites and CHT stromal cells ( Supplementary Fig. 6a–d ) but not in the fin mesenchymal cells ( Supplementary Fig. 6e ) in morphants relative to controls. Close inspection by combined VE-DIC and fluorescence microscopy did confirm the presence, only in the morphants, of stromal cells visible by VE-DIC that had virtually no more detectable mCherry signal ( Supplementary Fig. 6b , arrowheads). By 60–72 h.p.f., both fluorescence and VE-DIC microscopy evidenced a virtually complete lack of stromal cells in the naca morphant ( Fig. 6e,f , Supplementary Fig. 6f,g ). In parallel, the CV plexus was slightly thinner in the naca morphant at 48 h.p.f. and displayed fewer and often larger intervascular spaces in sagittal optical section ( Fig. 6c,d,h,i ). Between 48 and 60 h.p.f., these spaces flattened and the difference in CV plexus thickness between control and morphant larvae kept increasing ( Fig. 6e,f , Supplementary Movie 8 ), as observed above in the Tg[CD41:gfp] background ( Fig. 3e–h ). In addition, in the thinner naca morphant CHT, blood kept circulating in the various branches of the CV plexus, unlike in controls in which blood eventually flows only through the ventral-most branch, the definitive CV, as the more dorsal branches become packed with haematopoietic cells [6] . Both features thus are likely consequent to the lack of haematopoietic cells accumulation in the naca morphant CHT. NACA is cell-autonomously required for stromal cell survival Our data suggest naca deficiency affects stromal cells survival during CHT niche maturation. To further investigate whether the requirement for naca in stromal cell development is cell-autonomous, gastrula transplantation was performed to generate chimeric embryos, in which naca function is partially recovered or affected within the stromal cell population. At early gastrula stage (40% epiboly), cells located at the outer margin of the blastoderm (where mesoderm fates arise) of wild-type (control MO-injected) Tg[H2A-gfp] (ref. 24 ) embryos (which express nuclear GFP ubiquitously) were transplanted into naca MO-injected Tg[TCF:nls-mCherry] at the same stage and place ( Fig. 7a–d ). Reciprocally, cells from naca MO-injected Tg[H2A-gfp] embryos were transplanted in the same way into control MO-injected Tg[TCF:nls-mCherry] embryos ( Fig. 7e–h ). Recipient embryos were individually followed up at 42 and 60 h.p.f. At 42 h.p.f., SRCs originating from the wild-type H2A-GFP + donor could be observed in the naca morphant recipient in 7/120 successful transplants ( Fig. 7a,b ). These transplanted H2A-GFP + stromal cells had slightly expanded by 60 h.p.f., while the naca -deficient endogenous TCF:nls-mCherry + stromal cells had mostly disappeared ( Fig. 7c,d,i ). In the reciprocal experiment, cells transplanted from naca MO-injected H2A-GFP + donors into wt recipient Tg[TCF:nls-mCherry] embryos also provided stromal cells associated with the caudal plexus at 42 h.p.f., in 6/120 successful transplants ( Fig. 7e,f ); however their number had greatly decreased by 60 h.p.f., unlike the TCF:nls-mCherry + stromal cells from the wild-type recipient which had slightly expanded ( Fig. 7g,h,j ). These results demonstrate that naca is cell-autonomously required for SRC survival. 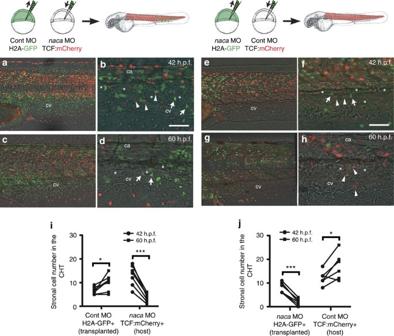Figure 7:nacais cell autonomously required for stromal cell survival during CHT maturation. (a–d) Cells at the ventral margin of control MO-injected H2A-GFP+embryos at 40% epiboly stage were transplanted into the same territory ofnacaMO-injected TCF:nls-mCherry embryos; a transplanted embryo is shown at 42 h.p.f. (a,b) and 60 h.p.f. (c,d); arrows and arrowheads indicate transplanted wild-type H2A-GFP+and endogenousnaca-deficient TCF:nls-mCherry+stromal cells, respectively. (e–h) Reciprocal experiment, transplanting cells fromnacaMO-injected H2A-GFP+embryos into control MO-injected TCF:nls-mCherry embryos; transplanted embryo at 42 h.p.f. (e,f) and 60 h.p.f. (g,h); arrows and arrowheads indicate transplantednaca-deficient H2A-GFP+and wild-type TCF:nls-mCherry+stromal cells, respectively. Asterisks indicate intervascular spaces within the developing CHT plexus typically harbouring stromal cells at these stages. (i,j) Quantification of CHT stromal cells of donor and recipient origin at 42 and 60 h.p.f. in the embryos that contained donor-derived CHT stromal cells at 42 h.p.f. Statistical significance determined using pairedt-test. *P<0.05, ***P<0.001. ca, caudal artery; cv, caudal vein. Scale bars, 50 μm. Figure 7: naca is cell autonomously required for stromal cell survival during CHT maturation. ( a – d ) Cells at the ventral margin of control MO-injected H2A-GFP + embryos at 40% epiboly stage were transplanted into the same territory of naca MO-injected TCF:nls-mCherry embryos; a transplanted embryo is shown at 42 h.p.f. ( a , b ) and 60 h.p.f. ( c , d ); arrows and arrowheads indicate transplanted wild-type H2A-GFP + and endogenous naca -deficient TCF:nls-mCherry + stromal cells, respectively. ( e – h ) Reciprocal experiment, transplanting cells from naca MO-injected H2A-GFP + embryos into control MO-injected TCF:nls-mCherry embryos; transplanted embryo at 42 h.p.f. ( e , f ) and 60 h.p.f. ( g , h ); arrows and arrowheads indicate transplanted naca -deficient H2A-GFP + and wild-type TCF:nls-mCherry + stromal cells, respectively. Asterisks indicate intervascular spaces within the developing CHT plexus typically harbouring stromal cells at these stages. ( i , j ) Quantification of CHT stromal cells of donor and recipient origin at 42 and 60 h.p.f. in the embryos that contained donor-derived CHT stromal cells at 42 h.p.f. Statistical significance determined using paired t -test. * P <0.05, *** P <0.001. ca, caudal artery; cv, caudal vein. Scale bars, 50 μm. Full size image NACA deficiency triggers the UPR and stromal cell apoptosis Previous reports have shown that NACA depletion can cause ER stress and ER stress-induced apoptosis through activation of the unfolded protein response (UPR) pathway in mammalian cultured cells [25] . We therefore analysed the expression of seven UPR-related genes in sibling and mutant larvae at 3.5 d.p.f. Four genes ( atf4 , bip , chop and xbp-1 ) coding for UPR effectors were significantly up-regulated in the mutant ( Fig. 8a ). In contrast, three genes ( atf6 , ire1 and perk ) encoding ER stress sensors showed little or no significant difference in expression between oloca mutant and sibling larvae ( Fig. 8b ). To clarify whether NACA-deficient cells may die by apoptosis, we performed whole mount TUNEL staining in oloca mutants in different transgenic backgrounds. By 3 d.p.f., TUNEL + signals were observed in the CHT of mutant but not sibling larvae. Using tyramide-amplified immunodetection, we could detect double positive, TCF:nls-mCherry + /TUNEL + apoptotic bodies, evidencing apoptotic death of TCF:nls-mCherry + mutant stromal cells ( Fig. 8c–e ). In contrast we found virtually no TUNEL + apoptotic bodies among gata1:DsRed + erythroid cells, mpx:GFP + neutrophils, CD41:GFP low HSPCs and ikaros:GFP + lymphoid progenitors in the mutant CHT ( Supplementary Fig. 7a–h ). 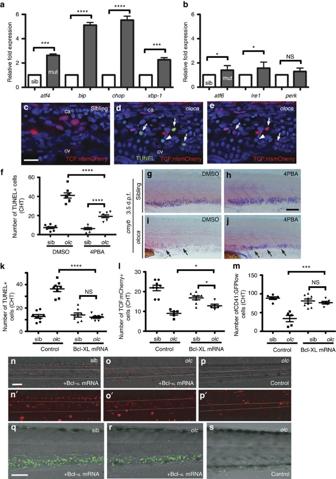Figure 8: NACA deficiency induces the unfolded protein response (UPR) and results in apoptosis. (a,b) qPCR reveals significant increase in transcript levels ofatf4,bip, chopandxbp-1(a) but not inatf6,ire1andperk(b) inolocamutants relative to siblings (n=3 biological replicates, average of 3 independent experiments). (c–e) TUNEL staining was performed onolocamutants and siblings at 3 d.p.f. in the TCF:nls-mCherry transgenic background. Arrows and arrowhead indicate TCF:nls-mCherry/TUNEL double positive cells and TUNEL single positive cells, respectively. (f) Number of TUNEL+cells in the CHT of control (DMSO)- or 4PBA-treatedolocamutant and sibling embryos at 3.5 d.p.f. (n=2 separate treatments). (g–j) WISH forcmybexpression in the CHT of control (DMSO) or 4PBA-treatedolocamutant and sibling embryos at 3.5 d.p.f. (k) Number of TUNEL+cells in the CHT of Bcl-XLmRNA injected or control embryos at 3.5 d.p.f. (n=2 separate injections). (l)in vivocounting of TCF:nls-mCherry+stromal cells in the CHT of Bcl-XLmRNA injected or control embryos at 60 h.p.f. (m–o'). (m)in vivocounting of CD41-GFPlowHSPCs in the CHT of Bcl-XLmRNA injected or control embryos at 3 d.p.f. (q–s).n=2 separate injections for (l) and (m). Error bars represent the s.d. and statistical significance determined using a Student’st-test. *P<0.05; ***P<0.001; and ****P<0.0001. n.s., not significant. Scale bars, 25 μm (c), 50 μm (n) and 100 μm (h,q). Figure 8: NACA deficiency induces the unfolded protein response (UPR) and results in apoptosis. ( a , b ) qPCR reveals significant increase in transcript levels of atf4 , bip, chop and xbp-1 ( a ) but not in atf6 , ire1 and perk ( b ) in oloca mutants relative to siblings ( n =3 biological replicates, average of 3 independent experiments). ( c – e ) TUNEL staining was performed on oloca mutants and siblings at 3 d.p.f. in the TCF:nls-mCherry transgenic background. Arrows and arrowhead indicate TCF:nls-mCherry/TUNEL double positive cells and TUNEL single positive cells, respectively. ( f ) Number of TUNEL + cells in the CHT of control (DMSO)- or 4PBA-treated oloca mutant and sibling embryos at 3.5 d.p.f. ( n =2 separate treatments). ( g – j ) WISH for cmyb expression in the CHT of control (DMSO) or 4PBA-treated oloca mutant and sibling embryos at 3.5 d.p.f. ( k ) Number of TUNEL + cells in the CHT of Bcl- XL mRNA injected or control embryos at 3.5 d.p.f. ( n =2 separate injections). ( l ) in vivo counting of TCF:nls-mCherry + stromal cells in the CHT of Bcl- XL mRNA injected or control embryos at 60 h.p.f. ( m – o '). ( m ) in vivo counting of CD41-GFP low HSPCs in the CHT of Bcl- XL mRNA injected or control embryos at 3 d.p.f. ( q – s ). n =2 separate injections for ( l ) and ( m ). Error bars represent the s.d. and statistical significance determined using a Student’s t -test. * P <0.05; *** P <0.001; and **** P <0.0001. n.s., not significant. Scale bars, 25 μm ( c ), 50 μm ( n ) and 100 μm ( h , q ). Full size image We then sought to block the ER stress/UPR pathway during CHT niche formation to determine whether activation of the UPR pathway causes stromal cell death and consequent defects in niche formation. Chemical chaperones such as 4-phenylbutyric acid (4-PBA) enhance protein folding and thus act as a suppressor of ER stress. When we treated oloca sibling and mutant embryos with 4-PBA, we found first that the fold enhancement of UPR genes ( atf4 , atf6 , bip and chop ) expression in mutant relative to sibling embryos was significantly decreased ( Supplementary Fig. 7i ); second, the number of TUNEL + cells was also decreased in the CHT of oloca mutants ( Fig. 8f ). Third, 4-PBA treatment significantly rescued the number of HSPCs marked by cmyb in situ hybridization at 3.5 d.p.f. ( Fig. 8g–j ). Finally, injection of mRNA encoding the anti-apoptotic protein Bcl- XL in oloca mutant embryos totally suppressed the occurrence of TUNEL + cells in the mutant CHT ( Fig. 8k ). It only partly rescued the number of TCF:nls-mCherry + stromal cells at 60 h.p.f. ( Fig. 8l,n–p ), possibly reflecting the faster extinction of the transgene in the mutant, and it fully rescued the number of CD41-GFP + HSPCs at 3 d.p.f., up to the wild-type level ( Fig. 8m,q–s ). We previously described that in zebrafish development, the CHT—the initial niche where definitive HSPCs home, expand and differentiate—consists of two main cell types: the venous endothelial cells of the CV plexus, and a cytomorphologically homogeneous stromal cell type which we named the FRCs, given their similarity in cytology and spatial organization to the FRCs of adult fish kidney marrow and mammalian bone marrow [6] . The origin of these FRCs was so far unknown. Here we have discovered that they originate from the ventral border of the caudal somites, through a typical EMT. Having now better described the development of these cells in vivo , we prefer to designate them as SRCs, as this name represents their two salient characteristics. Like NCCs after their EMT from the neural tube, the SRCs emigrate from the caudal somites as strings of cells that often divide on the way. They will constitute an excellent, readily accessible model for future in vivo studies of EMT. Although very little is known about the corresponding haematopoietic niche in mammals, in the fetal liver, Chagraoui et al . [26] reported that in vitro haematopoiesis-supportive stromal cells isolated from fetal liver consisted of ‘EMT cells’, as defined by co-immunostaining with a series of epithelial and mesenchymal markers. Recently, Nguyen et al . [27] demonstrated that trunk somites give rise to cells that incorporate in the DA and facilitate the hemogenic specification of other endothelial cells in the DA floor. Thus, our present work and this study together reveal an amazingly pervasive, and so far entirely unsuspected, cellular contribution of somite-derived cells in nurturing HSC development and then function, in first the specification of HSCs within the aorta [27] , and later their expansion and differentiation in the first niche where they home (this work). In the CHT, the ventral-wards emigration of SRC progenitors from the somite border closely accompanies the formation of the CV plexus in the same space, such that by 32–35 h.p.f., the very onset of HSPC budding from the aorta floor, the CV plexus is complete, with blood circulating through all its branches, and SRC progenitors interconnecting the CV branches. The niche is thus ready just in time to trap the first circulating aorta-derived HSPCs. Over the next 24 h, the SRC progenitors reorganize and mature into SRCs partly lining the abluminal face of the venous sinusoids. In mammals, neural crests contribute to bone marrow niche formation via nestin + mesenchymal stem cells [28] . In contrast, we observed no contribution of NCCs to the CHT other than pigment cells, and found normal SRCs and CHT haematopoiesis in a sox10 null mutant which lacks most neural crest derivatives. Here we could observe the mesenchymal SRC progenitors in vivo due to their labelling through a Wnt signalling reporter transgene. This does not necessarily imply that these cells keep receiving and transducing Wnt signals. Indeed, the TCF:GFP or TCF:nls-mCherry reporter is highly expressed in the somites and consequently in the SRC progenitors as they emerge from them, but then the fluorescent signal progressively decays in these cells, such that by 3 d.p.f., they are no longer detectable in vivo by this means, suggesting that the reporter protein was mostly inherited from the somitic origin. The second main result of our study is that a deficiency in NACA drastically compromises the sustainability and differentiation of HSPCs in the CHT, due to a defect not in the HSPCs, but in the CHT niche, making the oloca mutant the first of this kind in the zebrafish literature so far. In the oloca mutant, HSPCs, whether autologous or transplanted from wild-type adult kidney marrow home to the CHT niche just as in a wt larva, but then are unable to stay, expand and differentiate there. We traced this defect of the CHT niche to a defective maturation of the SRCs. Initially, SRC progenitors emerge normally from the somites, and accompany the formation of a functional CV plexus, which traps circulating HSPCs as well as in wild type. But then, over the next 2 days, the SRC progenitors progressively disappear instead of maturing into SRCs, and the resulting CHT is unable to support HSPC maintenance. We found that NACA is required cell autonomously for the maturation and survival of SRCs. Why does NACA deficiency cause the disappearance of SRC progenitors in particular? In mammals, NACA deficiency can cause ER stress and consequently the UPR, which, depending on the context, can trigger apoptosis [25] , [29] . We found that NACA deficiency does trigger the UPR in zebrafish larvae, and that treatment of naca mutants with the chemical chaperon 4-PBA significantly suppressed SRC apoptosis, and restored CHT haematopoiesis. Interestingly, EMT-derived mesenchymal cells in general were recently shown to be exquisitely sensitive to ER stress-induced apoptosis [30] . This feature was shown to be linked to their high level of extracellular matrix secretory activity, which involves steady ER development. Here in the CHT, the mesenchymal SRC progenitors are most likely responsible for secreting the large amount of extracellular matrix that surrounds the CV plexus by 48 h.p.f. [6] , which would render them more sensitive to the ER stress caused by NACA deficiency. Finally, the transplantation of WKM cells from adult fish into 2 d.p.f. larvae revealed an unexpected feature. The WKM cells readily homed not only to the CHT, but also to the kidney area. This was surprising because the developmental colonization of kidney by larval HSPCs only starts by 4 d.p.f. [6] , [31] . This unexpected observation suggests that developmentally, the kidney niche is potentially able to trap circulating HSPCs already by 2 d.p.f., but that larval HSPCs are not yet able to home to it. Now, whereas wild-type WKM cells similarly homed to the wt and oloca mutant kidney short after transplantation, 2 days later these cells had disappeared from the mutant kidney area, while they had expanded in the wild type. This observation suggests that NACA deficiency may affect not only the CHT niche, but also the kidney marrow niche, in a similar way. The early (pronephric) kidney niche has not been much studied yet, but similar SRCs are found in the CHT and adult kidney marrow niches [6] . Therefore we suggest that NACA deficiency may affect CHT and kidney marrow SRCs/FRCs in the same way, with similar consequences. The same may well apply to mesenchymal cells of mammalian haematopoietic niches such as the bone marrow. Zebrafish Transgenic and mutant stocks of zebrafish were raised and staged according to Westerfield [32] . AB wild-type fish and transgenic lines Tg[fli1:gfp] [33] , Tg[mpx:gfp] [34] , Tg[lysC:DsRed] [35] , Tg[lmo2:DsRed] [36] , Tg[gata1:DsRed] [37] , Tg[CD41:gfp] [38] , Tg[ikaros:gfp] [39] , Tg[TCF:gfp], Tg[TCF:nls-mCherry] [20] , Tg[H2A-gfp] [24] and sox10 cls m618 mutant [40] in Tg[sox10:egfp] [23] background were used. Generation and identification of the oloca mutant The oloca mutant (allele t30953 ) was identified in a large-scale N -ethyl- N -nitrosourea (ENU) mutagenesis screen (Tübingen 2005 Screen Consortium) by whole-mount Sudan Black staining of neutrophils [9] in 4 d.p.f. larvae. Meiotic mapping of oloca t30953 was performed using standard simple sequence length polymorphisms. The naca gene was cloned from cDNA made from mutant and wild-type siblings (primers nacaF1 and nacaR1). DNA was sequenced on both strands (primers nacaF2 and nacaR2). Genomic sequencing was performed by PCR amplification of naca exon 3 from mutant and wild-type larvae (primers nacaF3, nacaR3, nacaF4 and nacaR4). Primers used are listed in Supplementary Table 1 . The naca wild-type and mutant cDNAs were cloned into pCS2 + for mRNA injections (primers nacaF5 and nacaR5). In situ hybridization Whole-mount RNA in situ hybridization was performed according to Thisse ( https://wiki.zfin.org/display/prot/Thisse+Lab+-+In+Situ+Hybridization+Protocol+-+2010+update ) on embryos fixed at 26, 35, 48 and 72 h.p.f., 4 and 5 d.p.f. Riboprobes were synthesized for cmyb [41] , gata1 (ref. 42 ), ßE1-globin [43] , c/ebp1 (ref. 44 ), ikaros [45] , lck [46] , lysozyme C [47] , nephrosin (GenBank accession number. AY330223 ), csf1ra [48] . The naca wild-type cDNA cloned into pCS2 + vector was used for naca probe synthesis. Morpholino and mRNA injections One to two-cell-stage embryos were microinjected with 4 ng of a splice blocking antisense morpholino (MO) synthesized against naca ; naca MO1, 5′-TTAAAAGCAGTACTAACCCGTCTCA-3′, Genetools). Efficacy of MO knockdown was assessed by typical morphological abnormalities of oloca mutant and following SB staining. Parallel studies using another splice blocking MO ( naca MO2, 5′-AAAAGAAAGGCATCTTACCTGTGCC-3′) produced similar results, so all data presented in this study were derived from using naca MO1. For control embryos, the same amount of a standard control morpholino (5′-CCTCTTACCTCAGTTACAATTTATA-3′) was used. Wild-type and mutant mRNA used in the rescue assays were generated using the SP6 mMessage mMachine kit (Ambion) and co-injected with naca MO1 at a concentration of 125 ng μl −1 . Wide-field microscopy VE-DIC and fluorescence microscopy were performed as described previously [6] , [9] through the 60x/1.00 NA water-immersion objective of a Nikon 90i microscope. Time-lapse recording of VE-DIC images was performed using BTVpro software (Bensoftware, London). Bodipy ceramide staining Vital staining using Bodipy ceramide (Molecular probes) was performed as described previously [22] . Briefly, embryos at 19.5 h.p.f. were incubated in the staining solution (100 μM Bodipy ceramide, 2% dimethylsulphoxide (DMSO) in 10 mM HEPES (pH7.4)/E3 medium) for 30 min. at 28 °C. Embryos were rinsed in Volvic water and subjected to confocal microscopy. Confocal microscopy, image processing and quantification Confocal fluorescence microscopy was performed on Leica SPE and SP8 setups as described previously [18] . For quantification of the mean nls-mCherry fluorescence intensity per cell type in double Tg [TCF:nls-mCherry; Fli1:gfp] embryos, a volume of interest (VOI) was defined in 10 cells of each population of interest (stromal, somite muscle and fin mesenchymal cells) per embryo, and for each VOI the mean fluorescence/voxel was calculated using Imaris software (Bitplane). Eight control and eight naca MO-injected embryos were thus processed. The mean of 10 cells from each cell population was subjected to statistical analysis using unpaired two-tailed Student’s t -test (GraphPad Prism software). For nuclear tracking of Bodipy ceramide-stained TCF:nls-mCherry embryo, Imaris software was used for semiautomated four-dimensional tracking of nuclei over time; the tracks were manually checked under stereoscopic viewing, using Nvidia 3D-Vision glasses coupled to a double-frequency (120 Hz) video display. Whole kidney marrow transplantation Six adult Tg[mpx:gfp] transgenic fish were deeply anesthetized and all parts of the kidney (head, trunk and tail) were isolated in ice-cold PBS. WKM cells were prepared as described previously [49] . The cell suspension (5–8 × 10 5 ml −1 in PBS) of WKM was labelled with 5 μM of CellTracker Red CMTPX (Invitrogen) in PBS at 32 °C for 15 min, then washed several times in the zebrafish culture media previously reported by Stachura et al . [50] , then incubated at 32 °C for another 40 min to release excess CMTPX. Stained cells were prepared in the zebrafish culture media at a concentration of 5 × 10 7 ml −1 for the transplantation. Cell sorting for mpx-GFP + neutrophils was based on forward and side scatter and GFP fluorescence as described previously [37] , [51] , using a FACSAria III flow cytometer. Sorted mpx-GFP + cells were spun down and resuspended in DPBS (Invitrogen) at a concentration of 3 × 10 7 ml −1 for transplantation. CMTPX-labelled WKM cells or sorted mpx-GFP + cells were transplanted into 2 d.p.f. larvae (mutant or sibling) using the same setup as in Sarris et al . [52] . The cells were transplanted into the duct of Cuvier so as to enter circulation. Larvae with similar numbers of transplanted cells were kept overnight at 28 °C in E3 medium (5 mM NaCl, 0.15 mM KCl, 0.33 mM CaCl 2 , 0.33 mM MgSO 4 , methylene blue and 1-phenyl-2-thiourea, PTU). Two to thirty hours post transplantation larvae were mounted in 1% low melting point agarose in E3 medium supplemented with 0.16 mg ml −1 tricaine (Sigma) and used for imaging. Generation of parabiotic zebrafish embryos Four ng of naca MO or control MO were injected in 1-cell stage Tg[mpx:gfp] or Tg[lysC:DsRed] embryos, respectively. Injected morphants were raised until 1k-cell (late blastula) stage, then the two blastoderms were fused superficially as described [19] and let to develop into partially fused larvae. Non-injected Tg[mpx:gfp] and Tg[lysC:DsRed] embryos were fused for the control experiment. Transient expression of α-actin:GFP The plasmid p α act-GFPI2 containing skeletal muscle α- actin ( acta1a ) promoter driving GFP was co-injected with I-SceI meganuclease into 1-cell stage Tg[TCF:nls-mCherry] embryos (2.5–5 pg per embryo) as previously described [53] . Gastrula transplantation naca or control MO-injected embryos were dechorionated in a glass petri dish filled with high-calcium Ringer solution [19] at late blastula stage. Two donor ( naca or control MO-injected H2A-gfp) embryos and 4–5 host (control or naca MO-injected TCF:nls-mCherry) embryos were gently loaded using a glass pipet on a thin layer of 3% methylcellulose spread on a 30 mm petri dish filled with Ringer solution with antibiotics (penicillin/ streptomycin; 1% v/v). The transplant capillary was cut at 25 μm inner diameter and filled with Ringer solution before use. At 40% epiboly stage (5 h.p.f. ), ∼ 50–100 cells from the donor embryos were aspirated, targeting the ventral margin of the blastoderm that will give rise to somitic mesoderm, using the CellTram micromanipulator (Eppendorf). Around 50 cells were transplanted into the exact same location of each recipient embryo. The transplanted embryos were kept in the same solution overnight at 28 °C, then the medium was replaced with Volvic/PTU the next day. The number of GFP and nls-mCherry positive stromal cells in the CHT was counted at 42 and 60 h.p.f. for in each successfully transplanted recipient embryo. Statistical analysis was performed using paired t -test (GraphPad Prism software). 4-PBA treatment oloca mutant and sibling embryos were treated with 50 μM 4-phenylbutyrate (4-PBA; Sigma) in 10 mM HEPES (pH 7.4)/E3 medium from 24 h.p.f. The medium was renewed every day during the treatment period. Control embryos were incubated with vehicle (DMSO) alone at the equivalent concentration (0.01%). The 4-PBA- or DMSO-treated embryos were separated into sibling and mutant groups then fixed at 3.5 d.p.f. for in situ hybridization or TUNEL staining. Total RNAs for quantitative PCR (qPCR) analysis were extracted from groups of 15 oloca sibling or mutant embryos at 3.5 d.p.f. Bcl- XL mRNA injection For synthesis of Bcl- XL mRNA, the plasmid pCS2+flag-zBcl XL [54] was linearized with Not I then 1 μg of linearized plasmid was subjected to in vitro transcription using SP6 mMessage mMachine kit (Ambion). oloca mutant and sibling embryos in CD41:gfp or TCF:nls-mCherry transgenic background were injected with 200 pg of Bcl- XL mRNA per embryo at the one-cell stage. The injected embryos and non-injected controls were raised till 60 h.p.f. ( oloca :TCF:nls-mCherry) or 3 d.p.f. ( oloca :CD41:gfp), then subjected to confocal microscopy for cell counting. For the detection of oloca :TCF:nls-mCherry mutant embryos, confocal images of the CHT from 27 randomly chosen embryos were acquired at 60 h.p.f., and the embryos were then raised separately until 3 d.p.f. to ascertain their mutant or sibling phenotype. qPCR and TUNEL staining oloca sibling and mutant larvae were collected separately at 3–3.5 d.p.f. Total RNA was extracted using TRIzol reagent (Sigma) from each pool of 30 sibling and mutant embryos and 3 μg of total RNA were reverse transcribed to cDNA using M-MLV reverse transcriptase (Promega). Gene-specific primers were designed to detect an amplicon of each target gene of ∼ 150 bp. Each PCR reaction was performed with 10 ng cDNA using Power SYBR Green Master Mix (Life Technologies) and 250 nM of each primer. Primer sets used in this study are listed in Supplementary Table 2 . qPCR was carried out for three biological replicates with measurements taken from three technical replicates using a ABI7300 real-time PCR machine (Life Technologies). The relative expression of each gene was determined after being normalized to zebrafish elongation factor 1a ( ef1a ). Data in bars represent mean±s.d. Statistical analyses were performed using unpaired two-tailed Student’s t -test (GraphPad Prism software) and P values <0.001 were considered as significant. For the detection of apoptosis, oloca sibling and mutant embryos in various transgenic backgrounds were fixed at 3 d.p.f. in 4% methanol-free formaldehyde overnight then kept in methanol at −20 °C for at least 2 h. TUNEL staining was performed using ApopTag Red or Fluorescein In Situ Apoptosis Detection Kit (Chemicon) combined with peroxidase (POD) coupled anti-DIG antibody (Roche #11207733910, 1:200) followed by tyramide-based amplification [9] . To visualize the transgenic reporter proteins, rabbit anti-GFP (MBL #598, 1:300) or rabbit anti-DsRed/mCherry (Clontech #63296, 1:300) antibodies were co-incubated with the POD-coupled anti-DIG antibody, then revealed by anti-rabbit-AlexaFluor 488 (Life Technologies; #A11070, 1:200) and anti-rabbit-Cy3 (Jackson Lab; #711166152, 1:300) coupled antibodies, except for the [TCF:nls-mCherry] larvae, which were subjected to tyramide-based detection of POD-coupled anti-rabbit antibodies (Life Technologies #G21234, 1:300). How to cite this article: Murayama, E. et al . NACA deficiency reveals the crucial role of somite-derived stromal cells in haematopoietic niche formation. Nat. Commun . 6:8375 doi: 10.1038/ncomms9375 (2015).